Gram-scale synthesis of single-crystalline graphene quantum dots with superior optical properties Graphene quantum dots (GQDs) have various alluring properties and potential applications, but their large-scale applications are limited by current synthetic methods that commonly produce GQDs in small amounts. Moreover, GQDs usually exhibit polycrystalline or highly defective structures and thus poor optical properties. Here we report the gram-scale synthesis of single-crystalline GQDs by a facile molecular fusion route under mild and green hydrothermal conditions. The synthesis involves the nitration of pyrene followed by hydrothermal treatment in alkaline aqueous solutions, where alkaline species play a crucial role in tuning their size, functionalization and optical properties. The single-crystalline GQDs are bestowed with excellent optical properties such as bright excitonic fluorescence, strong excitonic absorption bands extending to the visible region, large molar extinction coefficients and long-term photostability. These high-quality GQDs can find a large array of novel applications in bioimaging, biosensing, light emitting diodes, solar cells, hydrogen production, fuel cells and supercapacitors. Graphene quantum dots (GQDs) have currently aroused increasing attention because of a myriad of alluring physicochemical properties and a wide range of potential applications [1] , [2] , [3] , [4] , [5] , [6] , [7] , [8] , [9] , [10] , [11] , [12] , [13] , [14] , [15] , [16] , [17] , [18] , [19] , [20] , [21] , [22] , [23] , [24] , [25] , [26] , [27] , [28] , [29] , [30] , [31] , [32] , [33] , [34] , [35] , [36] , [37] . Compared with conventional semiconductor quantum dots (QDs) such as CdX (X=S, Se, Te) and PbS, GQDs are more environmentally friendly, biocompatible and photostable. High-quality colloidal GQDs with excellent optical properties are highly desirable for solution-processable applications including bioimaging [13] , [15] , [16] , [20] , [26] , [27] , [28] , [29] , biosensing [25] , [30] , [31] , [32] , [33] , light emitting diodes (LEDs) [6] , [34] , solar cells [4] , [6] , [8] , [10] , [19] , [35] , [36] and photocatalysis [21] , [22] . Recently, chemical and electrochemical cutting routes have been developed to produce water-soluble colloidal GQDs [2] , [6] , [8] , [9] , [11] , [12] , [13] , [16] , [17] , [18] , [19] , [20] , [21] , [22] , [23] , [33] , [34] , [36] , [37] and derivatives (carbon dots [38] , [39] , [40] , [41] and graphene oxide nanoparticles [42] , [43] , [44] ) using carbon precursors from nanocarbons (graphene sheets [2] , [16] , [17] , [20] , [21] and carbon nanotubes [36] ) to bulk graphite [34] , [38] or counterparts such as artificial graphite [9] , [33] , carbon fibres [13] and coal [18] . In most cases, however, such cutting is less effective, and thus GQDs can only be produced in small amounts. Moreover, GQDs produced by cutting methods typically exhibit extremely poor optical properties [2] , [8] , [9] , [11] , [13] , [16] , [18] , [19] , [20] , [21] . For example, their absorption bands are merely within the UV region, even though their sizes increase from a few [2] , [8] , [11] , [13] , [16] , [18] , [19] , [20] , [21] to dozens [9] of nanometres. The weak visible absorption of GQDs may limit their applications in bioimaging, solar harvesting and LEDs. Furthermore, their fluorescent quantum yields (QY) are rather low (<15% in most cases), and thus they show low brightness and resolution when applied to bioimaging [13] , [15] , [16] , [26] , [27] , [28] , [29] . All these inferior optical performances are correlated with the vast existence of defect states in their polycrystalline or highly defective structures [17] , [24] , which inevitably form during the uncontrollable cutting processes. Apart from the top-down strategy, a bottom-up strategy has also been developed using various aromatic molecules [3] , [4] , [5] , [7] , [14] , [45] , [46] , [47] , [48] , [49] . A large number of polycyclic aromatic hydrocarbon (PAH) molecules have been employed to fabricate insoluble carbon materials such as artificial graphite, carbon films and graphene ribbons by high-temperature pyrolysis [45] , [46] , [47] , [48] or metal-catalysed surface fusion [49] . Progress has also been made in the synthesis of colloidal GQDs from small substituted benzene derivatives using multistep oxidative condensation reactions in organic solutions [3] , [4] , [5] , [14] . However, the large-scale applications of the colloidal GQDs are hindered by the rather complicated, harsh, environmentally unfriendly and high-cost synthetic procedures. For example, the organic-phase synthesis included 7–9 condensation steps performed under anhydrous and argon-protecting conditions, used many toxic and volatile organic solvents, and needed costly catalysts to drive the condensation reactions. Moreover, the GQDs were stabilized by three-dimensional (3D) cages composed of long phenyl moieties, which substantially modified the properties of the GQDs. For instance, the phenyl moieties made the GQDs non-biocompatible and may quench their fluorescence through resonance energy transfer. Besides, the insulating cage would hinder carrier transfer and thus make optoelectronic devices less efficient [4] . Here we report the gram-scale mass production of highly fluorescent water-soluble GQDs based on water-phase molecular fusion using cheap and low-toxicity pyrene (C 16 H 10 ) as the precursor. Pyrene and substituted derivatives such as 1,3,6-trinitropyrene consist of four peri-fused benzene rings with a unique carbon skeleton similar to the primitive cell of graphene, as shown in Scheme 1 . Our synthetic design was based on the controlled fusion or condensation of such graphene-cell molecules into single-crystalline GQDs. The synthesis involved the nitration of pyrene in nitric acid followed by hydrothermal treatment in alkaline aqueous solutions, where alkaline species play a crucial role in control over the size, edge functionalization (-OH, -NH 2 , and -NHNH 2 ) and optical properties of GQDs. Compared with the multistep organic-phase fusion [3] , [4] , [5] , [14] , the water-phase fusion is simpler, greener, milder, lower in cost and higher in overall product yield. Moreover, the resulting water-soluble GQDs are almost perfect single crystals whose edge sites are well-passivated by short electron-donating moieties rather than by long-chain, electron-accepting phenyl moieties. As a result, the high-quality colloidal QDs are expected to be superior to the oil-soluble GQDs by multistep fusion and to highly defective water-soluble GQDs by chemical or electrochemical cutting in terms of electronic, optical, optoelectronic and other properties. As an example, excellent optical properties are here demonstrated, such as highly efficient excitonic fluorescence, strong excitonic absorption bands even spanning the whole visible region, exceptionally large molar extinction coefficients and long-term photostability. Formation conditions of functionalized GQDs PAH molecules are highly stable, so their fusion into graphitized carbon materials under catalyst-free pyrolytic conditions requires high enough temperatures (>600 °C) to drive the elimination of hydrogen and graphitization [45] , [46] , [47] , [48] . In the case of the hydrothermal fusion of PAH molecules into single-crystalline GQDs reported here, only considerably low temperatures (90–200 °C) were needed. This low-temperature fusion was realized in alkaline aqueous solutions, where the presence of alkaline species enables the elimination of hydrogen, condensation or graphitization and edge functionalization. Before the alkaline hydrothermal treatment, pyrene was required to be nitrated into 1,3,6-trinitropyrene in hot HNO 3 (refs 50 , 51 , 52 ) ( Supplementary Note 1, Supplementary Figs 1–3 ). In two control experiments, both commercial pyrene and 1-nitropyrene were used to perform the same hydrothermal reaction in place of 1,3,6-trinitropyrene, but no carbon-like products were produced. This contrast indicates that 1,3,6-trinitropyrene is more active than pyrene and 1-nitropyrene towards the hydrothermal condensation reaction. The enhanced reaction activity of trinitropyrene can be related to three positively charged sites of NO 2 groups, which enable nucleophilic substitution reactions to occur with many alkaline species such as OH − , NH 3 and NH 2 NH 2 added to the hydrothermal media. The introduction of these alkaline species allows us to explore the mass production of water-soluble OH- and amine-functionalized GQDs. 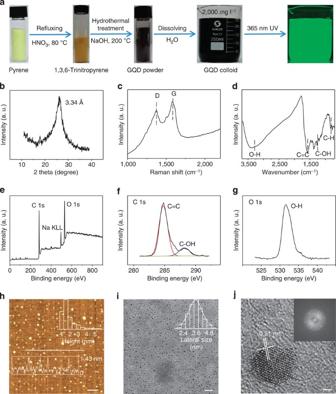Figure 1: Preparation and structural characterization of OH-GQDs. (a) Synthetic procedure. (b) XRD pattern. (c) Raman spectrum. (d) FT-IR spectrum. (e) Survey XPS spectrum. (f) High-resolution C 1 s spectrum. (g) High-resolution O 1 s spectrum. (h) AFM image (insets: height profile along the white line and height distribution). Scale bar, 500 nm. (i) TEM image (inset: lateral size distribution). Scale bar, 20 nm. (j) HRTEM image (Inset: FFT pattern). Scale bar, 1 nm. Hydroxyl-functionalized GQDs OH-functionalized GQDs (OH-GQDs) were typically synthesized by the nitration of pyrene in hot nitric acid at 80 °C followed by hydrothermal treatment in 0.2 M NaOH aqueous solution at 200 °C for 10 h. After the hydrothermal treatment, purification by dialysis, and drying at 80 °C, black OH-GQD powder (1.26 g) was obtained with an overall yield of 63% ( Supplementary Table 1 ). Resultant OH-GQDs can be redispersed in water with a high solubility of about 2,000 mg l −1 , and the dispersion or solution can keep stable for several months without precipitate ( Fig. 1a ). The OH-GQDs in aqueous solution emits bright green fluorescence when irradiated by a UV light (the sample is also denoted by g-GQDs) with a high QY of 23% (using Rhodamine 6G in ethanol as the reference). Their structure is characterized by X-ray powder diffraction (XRD), Raman, FT-IR (Fourier transform infrared) and XPS (X-ray photoemission spectroscopy) spectra. Its XRD pattern ( Fig. 1b ) is characteristic of graphite with a (002) layer spacing identical to that of bulk graphite (3.34 Å). The high graphitization is also shown in their Raman spectrum ( Fig. 1c ), where the ordered G band at 1,582 cm −1 is stronger than the disordered D band at 1,372 cm −1 with a large G to D intensity ratio of 1.2. Figure 1d shows the FT-IR spectrum of the dried OH-GQDs. A strong vibration at 1,590 cm −1 is ascribed to the C=C bonds, and a strong, rather broad vibration at ~3,400 cm −1 to the O-H bonds. Given that the sample has been fully dried just before the FT-IR test, the O-H signal is mainly ascribed to the hydroxyl functionalization of the GQDs, which is further confirmed by the vibration of C-OH at 1,270 cm −1 in the IR spectrum. The OH-functionalization of the GQDs is also revealed in the XPS spectra ( Fig. 1e–g ). The survey XPS spectrum ( Fig. 1e ) shows strong signals of C 1 s and O 1 s as well as a weak signal from impurity Na + . There is negligible N 1 s signal at ~400 eV. The high-resolution C 1 s spectrum ( Fig. 1f ) displays the strong signal of C=C at 284.8 eV and the distinguishable C-OH peak at 288.2 eV. The high-resolution O 1 s spectrum ( Fig. 1g ) reveals the presence of O-H at 531.4 eV. The XPS analysis demonstrates that 1,3,6-trinitropyrene is fused into OH-GQDs by total removal of the NO 2 group under the strongly alkaline hydrothermal conditions. The hydroxyl group is bonded with the single-crystalline GQD lattice most likely at edge sites rather than at basal plane sites. This unique edge-site functionalization could not induce any sp 3 defects within the graphene basal plane, which is different from random functionalization commonly observed in graphene oxide [42] , [43] , [44] and highly defective GQDs [2] , [11] , [12] , [13] , [16] , [17] , [18] , [19] , [20] , [21] , [22] , [23] , [33] , [34] , [36] , [37] cut from carbon materials. Their thicknesses characterized by atomic force microscope (AFM; Fig. 1h ) are largely in the range of 1 to 2 nm, with an average thickness of 1.47±0.86 nm, corresponding to an average layer number of ~5. Their transmission electron microscope (TEM) image ( Fig. 1i ) shows that the GQDs are well dispersed with uniform lateral sizes. Their average lateral size determined by TEM is 3.5±0.6 nm. Their typical atom-resolution structural imaging was taken by low-voltage aberration-corrected TEM ( Fig. 1j ). About 400 clearly distinguishable benzene rings are well arranged in a hexagonal honeycomb carbon network for a 4.5-nm GQD ( Fig. 1j ). This real-space image and its fast Fourier transform (FFT) pattern (inset in Fig. 1j ) show that the OH-GQDs are almost defect-free graphene single crystals with a spacing of 0.21 nm corresponding to that of graphene (100) planes. Figure 1: Preparation and structural characterization of OH-GQDs. ( a ) Synthetic procedure. ( b ) XRD pattern. ( c ) Raman spectrum. ( d ) FT-IR spectrum. ( e ) Survey XPS spectrum. ( f ) High-resolution C 1 s spectrum. ( g ) High-resolution O 1 s spectrum. ( h ) AFM image (insets: height profile along the white line and height distribution). Scale bar, 500 nm. ( i ) TEM image (inset: lateral size distribution). Scale bar, 20 nm. ( j ) HRTEM image (Inset: FFT pattern). Scale bar, 1 nm. Full size image Amine-functionalized GQDs The large-scale synthetic procedure of single-crystalline OH-GQDs can also be applied to the synthesis of amine-functionalized GQDs (amine-GQDs) by providing the amine functionalization with ammonia and hydrazine hydrate in the hydrothermal step. The large-scale synthesis of amine-GQDs in a 1,000-ml autoclave suggests that the commercial scale-up synthesis of single-crystalline GQDs is practical ( Supplementary Fig. 4 ). In ammonia solution, a colloid of yellow fluorescent, NH 2 -functionalized GQDs (y-GQDs) was yielded with a concentration of 1,600 mg l −1 ( Fig. 2a , right). Although there is a low fluorescence QY of 7%, their UV–vis absorption expands to the whole-visible region (Fig. 5a). In hydrazine hydrate solution, cyan fluorescent GQDs (c-GQDs) functionalized by NHNH 2 moiety with a high fluorescence QY of 26% were available. Under the coexistence of hydrazine hydrate and ammonia (4:1 molar ratio), the cyan fluorescence QY can be increased to 45%: the fluorescence under UV irradiation becomes brighter and dazzling when the colloid is diluted by 1,000 times ( Fig. 2a , middle). In the mixed alkaline solution, as the hydrothermal duration decreases from 10 to 1 h, blue fluorescent GQDs (b-GQDs) was also produced with a QY of 21% ( Fig. 2a , left). The AFM and TEM images of the three amine-GQD samples ( Fig. 2b,c ) show that the quantum dots in all the samples are uniform and well dispersed. The yellow, cyan and blue fluorescent GQDs have gradually decreasing average lateral sizes (3.8±0.5, 2.9±0.5, 2.6±0.6 nm), as expected by their different fluorescent colours that depend on the quantum confinement effect. Their average heights are 1.98±0.87, 0.81±0.39 and 1.07±0.51 nm, respectively. The thinnest c-GQDs most consist of 1–2 graphene layers. Their typical HRTEM images and FFT patterns are shown in Fig. 2d and Supplementary Figs 5 and 6 . The observation of the hexagonal honeycomb carbon networks and sixfold symmetrical FFT patterns indicates that these amine-GQDs are high-quality single crystals like OH-GQDs. Their high crystal quality is also exhibited by their Raman spectra ( Fig. 3a ), where the ordered G bands are all stronger than the disordered D bands. Note that the G to D intensity ratios of the b- and c-GQDs are significantly larger than that of the y-GQDs (1.14–1.20 versus 1.03), though the formers have smaller lateral sizes. This result indicates that both b- and c-GQDs as well as g-GQDs have fewer defects than y-GQDs and thus show higher PL QYs. The functionalization of these GQDs is characterized and analysed by FT-IR, XRD and XPS spectra. For the FT-IR spectra ( Fig. 3b ), the three dried amine-GQD samples show similar spectroscopic characteristics. Besides the C=C vibration at 1,590 cm −1 , there are N-H vibrations at 3,200 and 1,620 cm −1 , O-H vibration at ~3,400 cm −1 and C-OH vibration at 1,270 cm −1 . This result reveals that the GQDs synthesized in the presence of ammonia and/or hydrazine hydrate are co-functionalized by both amine and hydroxyl. This co-functionalization is also confirmed by the XPS spectra of the c-GQDs ( Fig. 3d ). The XPS survey spectrum gives N and O contents of the c-GQDs as high as 16.91 at% and 12.53 at%, respectively. The high-resolution C 1 s spectrum shows the signals of C=C at 284.7 eV, N-C at 286.1 eV and C-OH at 287.9 eV. The high-resolution N 1 s spectrum reveals the signals of NHNH 2 at 399.6 eV and N-C at 401.9 eV with atomic percent of 12.02 and 3.58%, respectively. The much lower atomic percent of N-C than that of NHNH 2 suggests that NH 2 NH 2 molecules are chemically bonded to the GQDs through monodentate rather than bidentate conjunction. The signal of NO 2 is also visible at 405.4 eV for N1s and at 532.9 eV for O 1 s, but its content is as low as 1.25 at%. These XPS results reveal that for the c- and b-GQDs synthesized in hydrazine hydrate solutions, edge sites are functionalized by OH and NHNH 2 groups. We speculate that the functionalization by the larger moiety (NHNH 2 ) should induce larger layer spacing than by smaller moieties of OH and NH 2 . Indeed, there is a nearly identical (002) layer spacing (3.44–3.49 Å) in the c- and b-GQDs functionalized by NHNH 2 , substantially larger than those of NH 2 - and OH-GQDs (3.34 Å) ( Fig. 3c ). We also note that there are much broader (002) reflection peaks in c- and b-GQDs than in y- and g-GQDs ( Figs 1b and 3c ). The enhanced (002) broadening of c- and b-GQDs can be correlated with the functionalization of NHNH 2 , which produces GQDs with fewer layer numbers and smaller lateral sizes. Moreover, the NHNH 2 functionalization can prevent small GQDs from stacking or aggregation to form large carbon particles during the drying process for the XRD test. 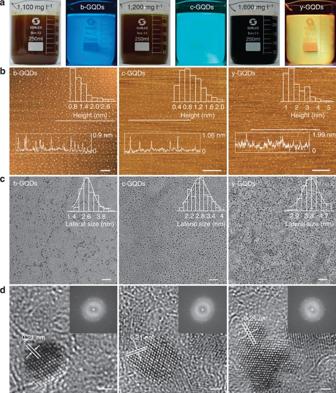Figure 2: Photographs of amine-GQDs. (a) Photographs of aqueous colloids of b-, c- and y-GQDs taken under UV (right) and visible (left) lights. (b) AFM images of b-, c- and y-GQDs (insets: height profiles along the white lines and height distributions). Scale bars, 2 μm, 500 nm and 2 μm, respectively. (c) Their TEM images (insets: lateral size distributions). Scale bar, 20 nm. (d) Their HRTEM images (insets: FFT patterns). Scale bar, 1 nm. Figure 2: Photographs of amine-GQDs. ( a ) Photographs of aqueous colloids of b-, c- and y-GQDs taken under UV (right) and visible (left) lights. ( b ) AFM images of b-, c- and y-GQDs (insets: height profiles along the white lines and height distributions). Scale bars, 2 μm, 500 nm and 2 μm, respectively. ( c ) Their TEM images (insets: lateral size distributions). Scale bar, 20 nm. ( d ) Their HRTEM images (insets: FFT patterns). Scale bar, 1 nm. 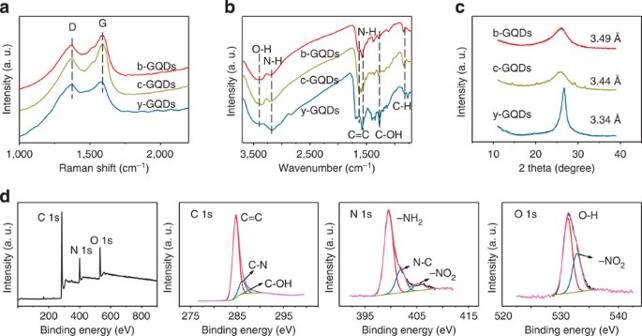Figure 3: Spectroscopic characterization of amine-GQDs. (a) Raman spectra of b, c- and y-GQDs. (b) Their FT-IR spectra. (c) Their XRD patterns. (d) XPS spectra of c-GQDs. Full size image Figure 3: Spectroscopic characterization of amine-GQDs. ( a ) Raman spectra of b, c- and y-GQDs. ( b ) Their FT-IR spectra. ( c ) Their XRD patterns. ( d ) XPS spectra of c-GQDs. Full size image Optical properties of single-crystalline GQDs Using highly fluorescent c-GQDs as a model, we systematically investigated the optical properties of single-crystalline GQDs. Their absorption spectrum (ABS in Fig. 4a ) exhibits three pronounced excitonic absorption bands centred at about 250, 290 and 400 nm, with an optical absorption edge at ~470 nm. They have a large molar extinction coefficient ( ε m ) of ~10 6 M −1 cm −1 within the visible region, even larger than that of conventional QDs (~10 5 M −1 cm −1 ) (ref. 53 ). Their PL peak at 475 nm can be excited in a wide wavelength range (PL, PLE in Fig. 4a ). The main PLE bands well agree with the corresponding excitonic absorption bands, suggesting that the emission is characterized by band-edge exciton-state decay rather than defect-state decay. This intrinsic PL characteristic is also exhibited in the PL decay curve ( Fig. 4b ), which shows monoexponential decay and one long lifetime (7.26 ns). Moreover, the PL maximum is well confined, nearly irrespective of excitation wavelength ( Fig. 4c ). All these superior optical characteristics and high PL yield (45%) are well correlated with the high-quality features of the GQDs such as almost defect-free single-crystalline structure and ideal electron-donating functionalization at edge sites rather than at basal plane sites. In marked contrast, previously reported GQDs usually exhibit poor optical properties [2] , [8] , [9] , [11] , [13] , [16] , [18] , [19] , [20] , [21] , which are related to their highly defective structures with a great number of sp 3 and vacancy defect states in the basal plane [17] , [24] . The photostability of the GQDs was tested under 3-h continuous radiation using a 100 W xenon lamp. The PL intensity and emission brightness of the GQDs are remarkably enhanced by the UV exposure ( Fig. 4d,e ). In a contrast test, conventional semiconductor QDs such as CdSe/ZnS core-shell QDs show a typical photobleaching effect that leads to the attenuation of their PL intensity and brightness on the UV exposure. This contrast clearly demonstrates that GQDs are more robust than the best protected compound semiconductor QDs. The PL enhancement may be ascribed to the UV-assisted replacement of remaining electron-accepting NO 2 groups by electron-donating OH groups at edge sites of the GQDs. To confirm the UV-induced substitution reaction, the c-GQDs treated by UV exposure for 3 h was further analysed by elemental analysis and XPS. Compared with the untreated sample, the H:N atomic ratio of the treated GQDs determined by elemental analysis increases from 3.26 to 5.03; The N and O molar contents determined by XPS decrease from 17.1 to 13.0% and from 13.4 to 9.7%, respectively. The H, N and O contents in the UV-treated sample are consistent with expected variations induced by substitution of remaining NO 2 groups for OH. Moreover, the high-resolution XPS spectra clearly show the absence of the NO 2 group at 405.4 eV in the N 1 s spectrum ( Supplementary Fig. 7c ) and the strong signal of the OH group at 531.3 eV in the O 1 s spectrum ( Supplementary Fig. 7d ). The PL stability of the GQDs was also tested in a wide range of pH values ( Fig. 4f ). The PL keeps relatively stable in neutral and basic solutions, but becomes markedly attenuated in strongly acidic media owing to the aggregation of the GQDs observed in acidic media. The optical properties of the c-GQDs were further investigated by varying synthetic conditions including nitration temperature and time, hydrothermal temperature and time, and alkali concentration. Their optical spectra show little variation when these parameters are changed ( Supplementary Figs 8 and 9 ), but the PL QY varies greatly ( Supplementary Table 2 ). 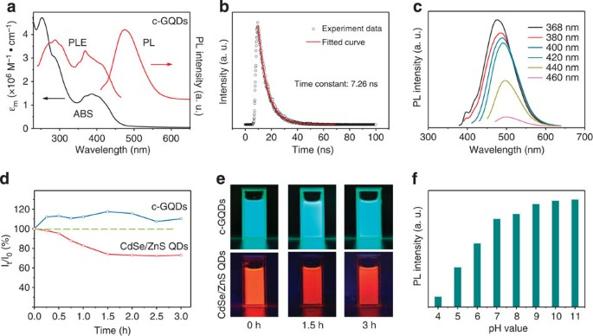Figure 4: Optical properties of c-GQDs. (a) UV-visible absorption (ABS), PL, and excitation (PLE) spectra. (b) Time-resolved PL spectrum. (c) PL spectra excited at different wavelengths. (d) Photostability comparison between c-GQDs and CdSe/ZnS QDs (Wuhan Jiayuan Co., Ltd.) under 365-nm UV light (100 W). (e) Digital photographs of c-GQDs and CdSe/ZnS QDs after the continuous irradiation of 0, 1.5, 3 h. (f) Dependence of PL intensity on pH values. Figure 4: Optical properties of c-GQDs. ( a ) UV-visible absorption (ABS), PL, and excitation (PLE) spectra. ( b ) Time-resolved PL spectrum. ( c ) PL spectra excited at different wavelengths. ( d ) Photostability comparison between c-GQDs and CdSe/ZnS QDs (Wuhan Jiayuan Co., Ltd.) under 365-nm UV light (100 W). ( e ) Digital photographs of c-GQDs and CdSe/ZnS QDs after the continuous irradiation of 0, 1.5, 3 h. ( f ) Dependence of PL intensity on pH values. Full size image It is of both scientific and technical significance to unveil size-dependent properties of novel QD systems. 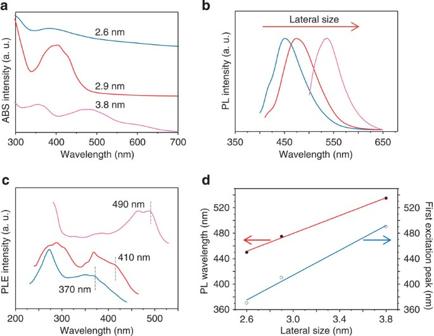Figure 5: Size-dependent optical properties of amine-GQDs. (a) Absorption spectra of GQDs with different average lateral sizes. (b) Their typical PL spectra. (c) Their typical PLE spectra (The first excitation peaks marked by dashed lines). (d) Dependence of PL wavelength and first excitation peak wavelength on lateral size. Figure 5 shows such size-dependent optical properties of single-crystalline amine-GQDs with different lateral sizes. For smaller b- and c-GQDs with lateral sizes of 2.6±0.6 and 2.9±0.5 nm, their absorption edges are near 450–470 nm ( Fig. 5a ). For larger y-GQDs of 3.8±0.5 nm, the excitonic absorption band extends from UV to the whole-visible region, with absorption edge near 650 nm. The PL wavelength of the GQDs increases with lateral size, as shown in Fig. 5b . The first excitation peak marked in the corresponding PLE spectra also shows the same trend with increasing lateral size ( Fig. 5c ). Linear size-dependent relationships of the PL wavelength and the first excitonic peak wavelength with the lateral size shown in Fig. 5d reveal the quantum confinement effect in colloidal single-crystalline GQDs. We also compare the optical properties of g- and y-GQDs with similar lateral sizes (3.5±0.6 nm for g-GQDs; 3.8±0.5 nm for y-GQDs) but with different functionalizations. Although the two kinds of GQDs are functionalized by OH and NH 2 , respectively, they show nearly the same optical characteristics in the UV–vis absorption, PL, PLE and pH-dependent PL spectra ( Supplementary Figs 10 and 11 ). There is only a slight redshift of PL wavelength for the y-GQDs relative to the PL of the g-GQDs. From all these results, it is concluded that the quantum confinement effect dominates the electronic and optical properties of the single-crystalline GQDs functionalized by these electron-donating groups. Figure 5: Size-dependent optical properties of amine-GQDs. ( a ) Absorption spectra of GQDs with different average lateral sizes. ( b ) Their typical PL spectra. ( c ) Their typical PLE spectra (The first excitation peaks marked by dashed lines). ( d ) Dependence of PL wavelength and first excitation peak wavelength on lateral size. Full size image Bright bioimaging of highly fluorescent GQDs Bestowed with superior optical properties such as high QYs, large molar extinction coefficients and long-term photostability, single-crystalline GQDs are expected to serve as excellent fluorescent probes for bioimaging. To evaluate this capability, 4T1 cells were cultured in a culture medium containing c-GQDs (10 mg l −1 ), and confocal microscopic images were taken using a 405-nm laser at a low voltage. Bright fluorescence observed in the whole cytoplasm area is ascribed to the internalized c-GQDs ( Fig. 6a,c ). The evidence for the internalization is given by z-axis imaging of the cells ( Supplementary Fig. 12 ). As the z-axis moves from the top to the bottom of the sample, the confocal cross-sectional images of individual cells become larger and brighter, and finally nearly invisible in turn. This observation indicates that the GQDs have been internalized by cells to the cytoplasm rather than bounded or adsorbed on the cell surface. Bright cell imaging was also taken on 488-nm laser excitation using green fluorescent GQDs internalized in 4T1 cells ( Fig. 6d,f ). The cellular toxicity of single-crystalline GQDs (c- and g-GQDs) was evaluated by CCK-8 viability assay. 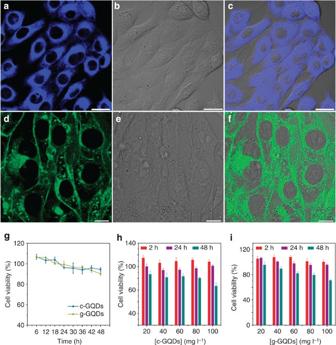Figure 6: Cell imaging and cytotoxicity assessment of GQDs using 4T1 cells. (a–c) Confocal fluorescence image (blue pseudocolour) at 405 nm excitation (a), bright field image (b) and merged image (c) of 4T1 cells using c-GQDs internalized into the cytoplasm of the cells. Scale bar, 20 μm. (d–f) Image (green pseudocolour) at 488 nm excitation (d), bright field image (e) and merged image (f) of 4T1 cells using g-GQDs. Scale bar, 10 μm. (g) Cell viability assays of c-GQDs and g-GQDs at the imaging dose (10 mg l−1) for incubation time varied from 6 to 48 h. (h) Cell viability assay of c-GQDs at higher doses. (i) Cell viability assay of g-GQDs at higher doses. Figure 6g shows the evolution of cell viability with incubation time at the imaging dose (10 mg l −1 ). The cell viability keeps over 90% for the two samples when the incubation time increases from 6 to 48 h, which is consistent with the observation of the increased living cell density with prolonging incubation time ( Supplementary Fig. 13 ). The dependence of the cell viability on GQD concentration is shown in Fig. 6h (c-GQDs) and Fig. 6i (g-GQDs). At concentrations of 20, 40, 60 and 80 mg l −1 , the cell viability is >80%, even though the incubation time is elongated to 48 h. These results indicate that both the amine- and OH-functionalized GQDs show no cytotoxicity at relatively high concentrations. When the concentration further increase to 100 mg l −1 and the incubation time is elongated to 48 h, the cell viability becomes below 80%, indicating of low cytotoxicity. However, the bright cell imaging can be realized at a GQD concentration (10 mg l −1 ) much lower than the toxic concentration (>80 mg l −1 ). Figure 6: Cell imaging and cytotoxicity assessment of GQDs using 4T1 cells. ( a – c ) Confocal fluorescence image (blue pseudocolour) at 405 nm excitation ( a ), bright field image ( b ) and merged image ( c ) of 4T1 cells using c-GQDs internalized into the cytoplasm of the cells. Scale bar, 20 μm. ( d – f ) Image (green pseudocolour) at 488 nm excitation ( d ), bright field image ( e ) and merged image ( f ) of 4T1 cells using g-GQDs. Scale bar, 10 μm. ( g ) Cell viability assays of c-GQDs and g-GQDs at the imaging dose (10 mg l −1 ) for incubation time varied from 6 to 48 h. ( h ) Cell viability assay of c-GQDs at higher doses. ( i ) Cell viability assay of g-GQDs at higher doses. Full size image We have developed a simple, green, low-cost and large-scale bottom-up approach for synthesizing OH- and amine-functionalized single-crystalline GQDs via alkali-mediated hydrothermal molecular fusion using an active PAH molecule as the precursor. Water-soluble single-crystalline GQDs offer outstanding optical properties such as strong excitonic absorption bands within the visible region, a large molar extinction coefficient, high PL QY, long-term photostability and less pH-dependent fluorescence. Therefore, single-crystalline GQDs provide higher-quality fluorescent probes for bioimaging than polycrystalline, less bright GQDs and conventional toxic and less photostable QDs. These GQDs can also find a large array of novel applications in light emitting diodes, solar cells, hydrogen production [22] , fuel cells [12] , [14] and supercapacitors [23] . Our findings will highlight the importance of large-scale aqueous growth for solution-processable single-crystalline graphene materials and exert a great impact on fluorescence microscopy for clinical diagnostic applications. Material synthesis In a typical procedure for synthesis of OH-GQDs, pyrene (2 g, TCI, purity >98%) was nitrated into trinitropyrene in hot HNO 3 (160 ml) at 80 °C under refluxing and stirring for 12 h. After cooled to room temperature, the mixture was diluted with deionized (DI) water (1 l) and filtered through a 0.22 μm microporous membrane to remove the acid. The resultant yellow 1,3,6-trinitropyrene (3.0 g, yield of 90%) was dispersed in an NaOH solution of DI water (0.6 l, 0.2 M) by ultrasonication (500 W, 40 kHz) for 2 h. The suspension was transferred to a poly(tetrafluoroethylene) (Teflon)-lined autoclave (1 l) and heated at 200 °C for 10 h. After cooled to room temperature, the product containing water-soluble GQDs was filtered through a 0.22 μm microporous membrane to remove insoluble carbon product, and further dialysed in a dialysis bag (retained molecular weight: 3,500 Da) for 2 days to remove sodium salt and unfused small molecules. The purified black OH-GQDs were dried at 80 °C for structural characterization and property measurement. The synthetic procedure of amine-GQDs was similar to that of the OH-GQDs except for the addition of different alkaline species in the media: 1.2 M ammonia for y-GQDs, 0.4 M ammonia and 1.5 M hydrazine hydrate for c- and b-GQDs. Material characterization AFM images were taken using a SPM-9600 AFM. TEM observations were performed on aberration-corrected TEM (FEI Titan 80–300) operating at 80 kV acceleration voltage, and a charge coupled device camera (2k × 2k, Gatan UltraScan 1000) was used for image recording with an exposure time of 1~2 s. XRD patterns were obtained with a Rigaku 18 KW D/max-2550 using Cu Kα radiation. Absorption and fluorescence spectra were recorded at room temperature on a Hitachi 3100 spectrophotometer and a Hitachi 7000 fluorescence spectrophotometer, respectively. FT-IR spectra of dried samples were recorded with a Bio-Rad FTIR spectrometer FTS165. Raman spectra were recorded on a Renishaw in plus laser Raman spectrometer with λ exc =785 nm. XPS spectra were collected using a Kratos Axis Ultra DLD X-ray photoelectron spectrometer. The PL QY of dilute b- and c-GQD aqueous solutions were determined by comparing the integrated PL intensities (excited at 400 nm) and the absorbency values (at 400 nm) using 9,10-bis(phenylethynyl) anthracene in cyclohexane (QY:100%) as the reference. The QYs of dilute g- and y-GQD aqueous solutions were determined by comparing the integrated PL intensities (excited at 490 nm) and the absorbency values (at 490 nm) using Rhodamine 6G (QY:95%) in ethanol as the reference. Cell imaging 4T1 cells were cultured in RPMI 1640 Formulation (1640) with L -glutamine (Gibco, USA), 10% (v/v) fetal bovine serum (Hyclone, USA). Approximately 2 × 10 5 4T1 cells were seeded in culture dishes (diameter: 40 mm) and cultured using the same culture medium (2 ml per dish) at 37 °C under 5% CO 2 /95% air. All cells were incubated for at least 24 h until ~80% confluence was reached. A GQD aqueous solution was introduced to the cells with a final concentration of ~10 mg l −1 in the culture medium. The cells were examined under a confocal microscope (Olympus FM 1000) using lasers of 405 and 488 nm. Cytotoxicity assay Cell viability assays were performed using a CCK-8Kit (Dojindo Laboratories, Japan) following the manufacturer’s instructions. The cell viability was expressed as the percentage of viable cells in total cells. 4T1 cells were seeded in 96-well plates (5 × 10 3 cells per well) and pre-cultured in medium containing the c- or g-GQDs at a dose of 10 mg l −1 for 6, 12, 18, 24, 32 and 48 h, respectively. The cell viability was further evaluated using higher GQD doses of 20, 40, 60, 80 and 100 mg l −1 for 2, 24 and 48 h. The cell viability of each well was treated with CCK-8 Kit following the manual, and the absorbance of each well at 450 nm was measured using a Microplate Reader (Thermo, USA). How to cite this article: Wang, L. et al . Gram-scale synthesis of single-crystalline graphene quantum dots with superior optical properties. Nat. Commun. 5:5357 doi: 10.1038/ncomms6357 (2014). The graphene lattice primitive cell (rhombus) consists of four peri-fused benzene rings identical to the carbon skeletons of pyrene and 1,3,6-trinitropyrene. More active 1,3,6-trinitropyrene with three positively charged sites tends to fuse into single-crystalline GQDs under base-assisting hydrothermal conditions.